Yes-associated protein regulates endothelial cell contact-mediated expression of angiopoietin-2 Angiogenesis is regulated by the dynamic interaction between endothelial cells (ECs). Hippo-Yes-associated protein (YAP) signalling has emerged as a key pathway that controls organ size and tissue growth by mediating cell contact inhibition. However, the role of YAP in EC has not been defined yet. Here, we show expression of YAP in the developing front of mouse retinal vessels. YAP subcellular localization, phosphorylation and activity are regulated by VE-cadherin-mediated-EC contacts. This VE-cadherin-dependent YAP phosphorylation requires phosphoinositide 3-kinase-Akt activation. We further identify angiopoietin-2 (ANG-2) as a potential transcriptional target of YAP in regulating angiogenic activity of EC in vitro and in vivo . Overexpression of YAP-active form in EC enhances angiogenic sprouting, and this effect is blocked by ANG-2 depletion or soluble Tie-2 treatment. These findings implicate YAP as a critical regulator in angiogenesis and provide new insights into the mechanism coordinating junctional stability and angiogenic activation of ECs. Angiogenesis is coordinated by the dynamics of quiescent and activated endothelial cells (EC) in response to multiple factors including growth factors, inflammatory cytokines or haemodynamic flow-induced mechanical forces [1] , [2] . Cell-to-cell junctions composed of adherens and tight junctions play important roles in maintaining the quiescence of ECs. It is conceivable that when ECs are activated by external or internal stimuli, the junctions become partially disorganized, and subsequent intracellular signalling induces cells to actively proliferate and migrate to form new vessels. Conversely, when actively proliferating ECs contact each other and form stable intercellular junctions, they become quiescent until the next signal arrives. Cell contacts, particularly in ECs, are significantly involved in endothelial barrier function and regulation of angiogenic remodelling as well as inhibition of cell proliferation [3] , [4] . Thus, EC junctions are more tightly regulated by extrinsic and intrinsic cellular changes, and in turn, ECs must delicately respond to junctional stability. VE-cadherin is a major EC-specific adherens junctional molecule that participates directly or indirectly in intracellular signalling to control cell dynamics or proliferation. VE-cadherin stabilizes the vasculature by associating with growth factor receptors, such as vascular endothelial growth factor receptor 2 and the transforming growth factor-β receptor, and regulating their activity [5] , [6] . VE-cadherin also influences cell dynamics by interacting with GTPase signalling, which is important in actomyosin contractility [7] . A recent study revealed that VE-cadherin is involved in the transcriptional regulation of genes, including claudin-5 (ref. 8 ). VE-cadherin-mediated cell–cell interaction activates the PI-3/Akt pathway, leading to phosphorylation and inactivation of FoxO1 transcriptional repressor, which results in upregulation of claudin-5 (ref. 8 ). Beta-catenin or p120 associated with VE-cadherin in adherens junctional complexes also translocates to the nucleus and activates the target genes in response to permeability-inducing factors [9] . These studies suggest that VE-cadherin-mediated cell adhesion is important for balancing the quiescent and active status of ECs. Angiogenic activation induced by vascular endothelial growth factor, inflammatory cytokines or haemodynamic flow changes leads to angiopoietin-2 (ANG-2) gene expression [10] . ANG-2 was first identified as a natural antagonist of ANG-1/Tie-2 signalling in ECs [11] . However, subsequent studies report conflicting results demonstrating its pro-angiogenic activity in vitro or in vivo [12] , [13] . ANG-2 also sensitizes ECs to respond to inflammatory cytokines, such as tumour-necrosis factor-α, and thus enhances angiogenesis triggered by inflammation [14] . Despite the controversy over its role in angiogenesis, most studies so far suggest that ANG-2 is relatively highly expressed at the active sites of vascular remodelling and plays a key role in controlling endothelial remodelling and angiogenesis [10] . Although the functional significance of its activity in endothelial homeostasis is well recognized, the mechanisms regulating ANG-2 expression remain undefined. Yes-associated protein (YAP) is a transcriptional co-activator that plays key roles in the contact inhibition of cell growth and organ size restriction [15] . Cytoplasmic localization of YAP is promoted through its phosphorylation by the Hippo kinase cascade, whose components and function are well conserved in mammals. Recently, YAP activity was shown to be regulated by cellular mechanical stress as well as cell–cell contact [16] , [17] . Considering the importance of mechanical stress and cell–cell contact in the regulation of vascular homeostasis, it is expected that YAP may play an important role in EC function. Nevertheless, the role of YAP in ECs has not been studied so far. Here, we show for the first time that YAP activity and nuclear localization are regulated by EC adherens junction protein, VE-cadherin-mediated cell contact. Furthermore, YAP increases ANG-2 expression and regulates endothelial function in vitro . YAP is expressed in the ECs of the neovascular region The regulation of YAP transcriptional activity and subcellular localization has been investigated largely in epithelial or tumour cells. To define the role of YAP in the vasculature, we first examined the expression pattern of YAP in mouse retinal vessels and human umbilical vein endothelial cells (HUVECs). Increased expression of YAP was detected in the front region of the retinal vessel at an early stage of development (postnatal day [P]5) and in the region of vessels invading into the internal layer (P8, P12), in which vascular junctions are dynamically regulated ( Fig. 1a,b and Supplementary Fig. 1a,b ). Interestingly, YAP was partially localized in the nuclei of ECs of the front vascular region at P5, whereas YAP was localized in the cytosol of ECs of the central region of the retinal vessels ( Fig. 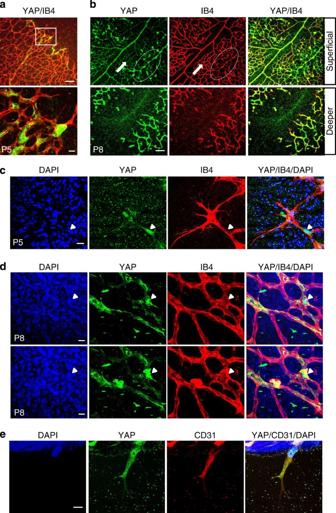Figure 1: Expression of YAP in mouse retinal vessels and endothelial sprouts from aortic rings. (a,b) Mouse retinas were prepared at postnatal day 5 or 8 (P5 or P8). Vessels were co-stained with the anti-YAP antibody (Green) and isolectin B4 (IB4; Red). (a) YAP staining in P5 retinal vessels. Scale bars, 100 μm (upper) and 20 μm (lower). (b) YAP expression in the developing retinal vessels at P8. The white arrow and dotted circle indicate relatively low or high YAP expression, respectively. Upper panels indicate the superficial layer, and lower panels indicate the deeper layer of the retinal vessel. Scale bar, 100 μm. (c) Immunofluorescence staining of nuclear localized YAP in mouse retinal vessels at P5. Scale bar, 20 μm. (d) Immunofluorescence staining of nuclear localized YAP at P8 mouse retinal vessel. Two different z-stacks were shown. White arrow heads indicate nuclear staining. Scale bar, 20 μm. Green: YAP, red: isolectin B4 (IB4), blue: DAPI. Six retinas per group were used for staining. (e) Nuclear YAP in endothelial sprouts emigrated from the mouse aortic ring. Scale bar, 20 μm. Green: YAP, red: CD31, blue: DAPI. 1c and Supplementary Fig 1c,d ). YAP was also detected in the nuclei of the invading retinal vessels at the branching points at P8 ( Fig. 1d and Supplementary Fig. 2a ). Nuclear localization of YAP in invading retinal vessels was confirmed by co-staining with antibodies against YAP and the EC nuclear marker, Erg 1/2/3 ( Supplementary Fig. 2b ). Nuclear YAP was also observed in endothelial sprouts that had just emigrated from aortic rings ( Fig. 1e ), suggesting that nuclear YAP may contribute to endothelial activation and sprouting. Furthermore, YAP was upregulated during endothelial differentiation from endothelial progenitor cells and remained highly expressed during HUVEC tube formation on Matrigel ( Supplementary Fig. 3 ), implying its important role in EC function. Figure 1: Expression of YAP in mouse retinal vessels and endothelial sprouts from aortic rings. ( a , b ) Mouse retinas were prepared at postnatal day 5 or 8 (P5 or P8). Vessels were co-stained with the anti-YAP antibody (Green) and isolectin B4 (IB4; Red). ( a ) YAP staining in P5 retinal vessels. Scale bars, 100 μm (upper) and 20 μm (lower). ( b ) YAP expression in the developing retinal vessels at P8. The white arrow and dotted circle indicate relatively low or high YAP expression, respectively. Upper panels indicate the superficial layer, and lower panels indicate the deeper layer of the retinal vessel. Scale bar, 100 μm. ( c ) Immunofluorescence staining of nuclear localized YAP in mouse retinal vessels at P5. Scale bar, 20 μm. ( d ) Immunofluorescence staining of nuclear localized YAP at P8 mouse retinal vessel. Two different z-stacks were shown. White arrow heads indicate nuclear staining. Scale bar, 20 μm. Green: YAP, red: isolectin B4 (IB4), blue: DAPI. Six retinas per group were used for staining. ( e ) Nuclear YAP in endothelial sprouts emigrated from the mouse aortic ring. Scale bar, 20 μm. Green: YAP, red: CD31, blue: DAPI. Full size image YAP is required for EC function in vitro and ex vivo To determine the effect of YAP on EC function and vascular remodelling, we knocked down YAP in ECs using short interfering RNA (siRNA) and performed tubular network formation and fibrin gel bead assays. YAP expression was efficiently reduced in siRNA-transfected HUVECs ( Fig. 2a ). YAP knockdown resulted in the defective tubular network formation of ECs on Matrigel ( Fig. 2b,c ). The reduction in YAP also suppressed sprouting from EC-coated beads in the fibrin gel ( Fig. 2d,e ). To further evaluate the effect of YAP on endothelial sprouting, we transfected mouse aortic rings with Yap-specific siRNA. Similar to the bead-assay results, Yap siRNA-transfected aortic rings displayed less sprouting ( Fig. 2f–h ). However, the viability and proliferation of ECs were not significantly affected by YAP knockdown ( Supplementary Fig. 4 ). Overall, these data demonstrate that YAP is critical for EC functions that are important in angiogenic sprouting and remodelling. 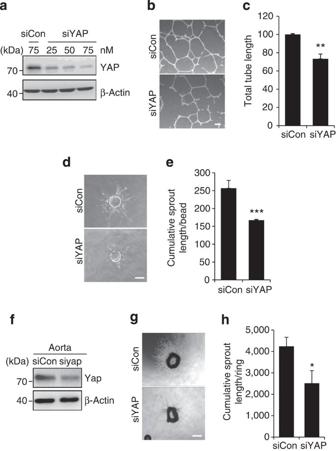Figure 2: YAP-deficient ECs display impaired angiogenic function. (a) Western blot analysis of YAP in HUVECs that were transfected with control siRNA (siCon) or increasing concentrations of YAP siRNA (siYAP). (b–e) HUVECs were transfected with 50 nM control or YAP siRNA. (b,c) The tubular network-forming activity of HUVECs was analysed on Matrigel. Representative tubular networks that formed (b) and the quantification of tube length are shown (c). Scale bars, 100 μm (d,e) Fibrin gel bead sprouting assay was performed and representative spheroids are shown for each condition (d) and cumulative sprout length derived from a bead was counted after 6 days incubation (e). Beads in 25 randomized microscopic fields were counted in each condition. Scale bars, 100 μm. (f–h) Sprouting from murine aortic rings were analysed in fibrin gel. (f) Aortic rings transfected with control or Yap siRNA (100 nM) were lysed, and Yap expression was detected by western blotting. (g) Representative aortic rings embedded in fibrin gel are shown. Scale bars, 100 μm. (h) Cumulative sprout length derived from aortic rings was quantified after 6 days incubation in the presence of bFGF. At least eight aortic rings were counted in each condition. Data show representative results from three independent experiments. Data are the means±standard error of the mean (s.e.m.) of values from a representative result. *P<0.05, **P<0.01, ***P<0.0001 (two-tailed Student’st-test). Figure 2: YAP-deficient ECs display impaired angiogenic function. ( a ) Western blot analysis of YAP in HUVECs that were transfected with control siRNA (siCon) or increasing concentrations of YAP siRNA (siYAP). ( b – e ) HUVECs were transfected with 50 nM control or YAP siRNA. ( b , c ) The tubular network-forming activity of HUVECs was analysed on Matrigel. Representative tubular networks that formed ( b ) and the quantification of tube length are shown ( c ). Scale bars, 100 μm ( d , e ) Fibrin gel bead sprouting assay was performed and representative spheroids are shown for each condition ( d ) and cumulative sprout length derived from a bead was counted after 6 days incubation ( e ). Beads in 25 randomized microscopic fields were counted in each condition. Scale bars, 100 μm. ( f – h ) Sprouting from murine aortic rings were analysed in fibrin gel. ( f ) Aortic rings transfected with control or Yap siRNA (100 nM) were lysed, and Yap expression was detected by western blotting. ( g ) Representative aortic rings embedded in fibrin gel are shown. Scale bars, 100 μm. ( h ) Cumulative sprout length derived from aortic rings was quantified after 6 days incubation in the presence of bFGF. At least eight aortic rings were counted in each condition. Data show representative results from three independent experiments. Data are the means±standard error of the mean (s.e.m.) of values from a representative result. * P <0.05, ** P <0.01, *** P <0.0001 (two-tailed Student’s t -test). Full size image YAP activity is regulated by endothelial cell–cell contact The transcriptional activity of YAP is known to be regulated by phosphorylation-dependent shuttling between the nucleus and the cytoplasm. YAP phosphorylation on S127 is enhanced by increased EC density ( Fig. 3a ), which is consistent with previous results in other cell types [17] . In sparse cell cultures, most YAP protein was localized to the nucleus of HUVECs, whereas YAP was localized to the cytoplasm of confluent HUVECs ( Fig. 3b ). Cellular fractionation experiments also revealed that YAP was localized to the cytoplasm and the nucleus of confluent and sparse cells, respectively ( Fig. 3c ). Furthermore, large amounts of YAP were phosphorylated in the cytoplasm of confluent cells, whereas no significant phosphorylation occurred in sparse cells ( Fig. 3c ). Accordingly, the expression of known target genes of YAP, including CTGF, ANKRD and Cyr61, was decreased in confluent cells ( Fig. 3d ). Interestingly, cells migrating from the scratch of confluent cells showed nuclear YAP staining in contrast to the cytoplasmic localization in non-migrating contacted cells ( Fig. 3e ). Transcriptional enhancer activator (TEA) domain protein (TEAD) is a major transcription factor that is bound and activated by YAP [18] . The nuclear activity of YAP, which was detected by using a luciferase reporter under the control of eight consecutive TEAD-binding sites, was controlled by EC density ( Fig. 3f ). Junctional breakage induced by EGTA [19] and the vascular permeability factor, thrombin [20] , also promoted nuclear localization of YAP in confluent ECs ( Supplementary Figs 5 and 6 and Fig. 3g,h ). In agreement with this, YAP phosphorylation was decreased by thrombin treatment ( Fig. 3i ). The luciferase activity of the YAP reporter and YAP-dependent gene expression were also increased by thrombin or EGTA ( Fig. 3j,k and Supplementary Fig. 6b ). It is noteworthy that YAP phosphorylation was not decreased by thrombin or EGTA treatment in sparsely cultured ECs ( Supplementary Fig. 6c ), which had little cell–cell contact. Thus, it is likely that the effects of thrombin or EGTA on YAP phosphorylation and activity are derived from the breakage of cell contacts rather than direct signalling effects. These results altogether suggest that EC contacts control the subcellular localization and transcriptional activity of YAP. 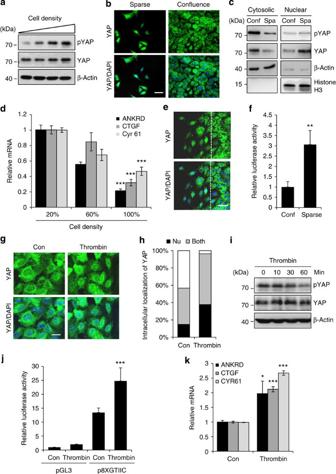Figure 3: YAP is phosphorylated and redistributed in a cell contact-dependent manner in ECs. (a) HUVECs were seeded at different cell densities in 60-mm plates. After 24 h, pYAP (S127) and YAP were determined by immunoblotting. Phosphorylation of YAP S127 residue was increased in a cell density-dependent manner. (b) HUVECs were sparsely or densely seeded on gelatin-coated coverslips in 12-well plates. Endogenous YAP was stained using anti-YAP antibody. Green: YAP, blue: DAPI. Scale bar, 50 μm. (c) HUVECs were cultivated as confluent (Conf) or sparse (Spa) cultures. The cytosolic or nuclear fraction of cell lysates was probed with anti-YAP or anti-phospho-YAP (S127). (d) Total RNA was extracted from HUVECs cultured in different densities, and relative RNA level of ANKRD, CTGF and Cyr61 were determined by semi-quantitative reverse transcription–PCR. (e) HUVECs were cultured under dense conditions and scratched. Cells were stained with anti-YAP antibody and DAPI 4 h after wounding. The dashed line indicates the original scratch. Green: YAP, blue: DAPI. Scale bar, 50 μm. (f) The luciferase activity of the TEAD-binding site containing the reporter (p8XGTIIC) was measured in confluent or sparse HUVECs. (g,h) Confluent cells were starved for 1 h and treated with 1 U ml−1thrombin for 1 h. (g) Cells were stained with YAP antibody (green) and DAPI (blue). Scale bar, 20 μm. (h) YAP localization was quantified. Nu, Both, and Cyto indicate the nuclear, both nuclear- and cytoplasmic-, and cytoplasmic-localized YAP, respectively. (i) Cell lysates from HUVECs treated with thrombin for indicated time were probed with antibodies against phospho-YAP (S127), YAP or β-actin. (j) HUVECs were transfected with pGL3-basic- or p8XGTIIC-Luciferase reporter along with pRL-Tk internal control vector. Cells cultured under confluent conditions were starved for 1 h and stimulated with thrombin for 1 h. Luciferase activity was measured and normalized to Renilla activity. (k) Densely cultured HUVECs were treated with 1 U ml−1thrombin for 4 h. Relative level of ANKRD, CTGF and Cyr61 transcript was determined. Data are means±standard deviation (s.d.) of triplicates; **P<0.01, ***P<0.0001 (two-tailed Student’st-test). Figure 3: YAP is phosphorylated and redistributed in a cell contact-dependent manner in ECs. ( a ) HUVECs were seeded at different cell densities in 60-mm plates. After 24 h, pYAP (S127) and YAP were determined by immunoblotting. Phosphorylation of YAP S127 residue was increased in a cell density-dependent manner. ( b ) HUVECs were sparsely or densely seeded on gelatin-coated coverslips in 12-well plates. Endogenous YAP was stained using anti-YAP antibody. Green: YAP, blue: DAPI. Scale bar, 50 μm. ( c ) HUVECs were cultivated as confluent (Conf) or sparse (Spa) cultures. The cytosolic or nuclear fraction of cell lysates was probed with anti-YAP or anti-phospho-YAP (S127). ( d ) Total RNA was extracted from HUVECs cultured in different densities, and relative RNA level of ANKRD, CTGF and Cyr61 were determined by semi-quantitative reverse transcription–PCR. ( e ) HUVECs were cultured under dense conditions and scratched. Cells were stained with anti-YAP antibody and DAPI 4 h after wounding. The dashed line indicates the original scratch. Green: YAP, blue: DAPI. Scale bar, 50 μm. ( f ) The luciferase activity of the TEAD-binding site containing the reporter (p8XGTIIC) was measured in confluent or sparse HUVECs. ( g , h ) Confluent cells were starved for 1 h and treated with 1 U ml −1 thrombin for 1 h. ( g ) Cells were stained with YAP antibody (green) and DAPI (blue). Scale bar, 20 μm. ( h ) YAP localization was quantified. Nu, Both, and Cyto indicate the nuclear, both nuclear- and cytoplasmic-, and cytoplasmic-localized YAP, respectively. ( i ) Cell lysates from HUVECs treated with thrombin for indicated time were probed with antibodies against phospho-YAP (S127), YAP or β-actin. ( j ) HUVECs were transfected with pGL3-basic- or p8XGTIIC-Luciferase reporter along with pRL-Tk internal control vector. Cells cultured under confluent conditions were starved for 1 h and stimulated with thrombin for 1 h. Luciferase activity was measured and normalized to Renilla activity. ( k ) Densely cultured HUVECs were treated with 1 U ml −1 thrombin for 4 h. Relative level of ANKRD, CTGF and Cyr61 transcript was determined. Data are means±standard deviation (s.d.) of triplicates; ** P <0.01, *** P <0.0001 (two-tailed Student’s t -test). Full size image VE-cadherin is critical for control of YAP activity in EC Stable EC junctions are very important in maintaining vascular integrity and homeostasis. Abnormality of peripheral blood vessel integrity is intimately related to several pathological conditions, including inflammatory diseases and cancer. The EC junction is mediated by homophilic linkage between adherens junction or tight junction protein complexes. VE-cadherin is a major protein of adherens junctions in ECs and is involved in multiple intracellular signalling pathways that regulate EC growth, survival and activation. VE-cadherin knockdown using specific siRNA in ECs reduced YAP phosphorylation and increased its nuclear localization ( Fig.4a–d and Supplementary Fig. 7a ). Furthermore, YAP transcriptional activity and YAP target gene expression were also increased by VE-cadherin reduction in ECs ( Fig. 4e,f ). The disruption of VE-cadherin-mediated cell–cell interaction using neutralizing VE-cadherin antibody led to reduction of YAP phosphorylation and nuclear localization ( Fig. 4g–j ). Consistently, the transcription of YAP-dependent genes was increased ( Fig. 4k ). Moreover, knockdown of β-catenin or α-catenin, which are components of the VE-cadherin junctional complex, reduced YAP phosphorylation in densely cultured ECs ( Supplementary Fig. 7b,c ), suggesting that formation of the VE-cadherin-mediated cell junctional complex is required for cell density-dependent YAP phosphorylation and localization. 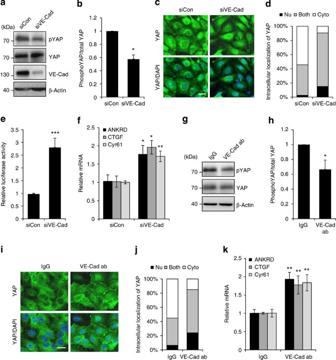Figure 4: VE-cadherin regulates cell contact-dependent YAP activity in ECs. (a,b) HUVECs were transfected with control siRNA (siCon) or VE-cadherin siRNA (siVE-Cad) and cultured under confluent conditions for 40 h. Cells were starved for 8 h, and cell lysates were probed with anti-pYAP, YAP, VE-cadherin (VE-Cad) or β-actin antibody. Phosphorylated YAP was quantified and normalized to YAP. (c,d) HUVECs were cultured under the conditions described ina,b. Cells were stained with anti-YAP antibody (green) and DAPI (blue), and the subcellular localization of YAP was quantified. Scale bar, 20 μm. (e) HUVECs were co-transfected with p8X GTIIC-luciferase reporter (1 μg) and control or VE-Cad siRNA (50 nM). Cells were cultured under the condition described ina. Luciferase activity was measured and normalized to internal control Renilla luciferase activity. (f) Densely cultured HUVECs were transfected with siRNA (50 nM) of VE-Cad. Relative level of ANKRD, CTGF and Cyr61 transcript was determined. (g,h) Densely cultured HUVECs were treated with neutralizing VE-cadherin antibody (VE-Cad ab; CAD5, 5 μg ml−1) for 6 h. Total cell lysates were analysed by western blotting for phosphorylated and total YAP expression using specific antibodies. The graph represents western blot quantification. (i) Immunofluorescence analysis of YAP in VE-Cad antibody-treated HUVECs. (j) Intracellular localization of YAP was quantified. Scale bar, 20 μm. Green: YAP, blue: DAPI. (k) Densely cultured HUVECs were treated with VE-cadherin antibody (5 μg ml−1). Relative level of ANKRD, CTGF and Cyr61 transcript was determined. Data are means±s.d. of triplicates. *P<0.05, **P<0.01, ***P<0.001 (two-tailed Student’st-test). Nu, Both, and Cyto indicate the nuclear, both nuclear- and cytoplasmic-, and cytoplasmic-localized YAP, respectively. Figure 4: VE-cadherin regulates cell contact-dependent YAP activity in ECs. ( a , b ) HUVECs were transfected with control siRNA (siCon) or VE-cadherin siRNA (siVE-Cad) and cultured under confluent conditions for 40 h. Cells were starved for 8 h, and cell lysates were probed with anti-pYAP, YAP, VE-cadherin (VE-Cad) or β-actin antibody. Phosphorylated YAP was quantified and normalized to YAP. ( c , d ) HUVECs were cultured under the conditions described in a , b . Cells were stained with anti-YAP antibody (green) and DAPI (blue), and the subcellular localization of YAP was quantified. Scale bar, 20 μm. ( e ) HUVECs were co-transfected with p8X GTIIC-luciferase reporter (1 μg) and control or VE-Cad siRNA (50 nM). Cells were cultured under the condition described in a . Luciferase activity was measured and normalized to internal control Renilla luciferase activity. ( f ) Densely cultured HUVECs were transfected with siRNA (50 nM) of VE-Cad. Relative level of ANKRD, CTGF and Cyr61 transcript was determined. ( g , h ) Densely cultured HUVECs were treated with neutralizing VE-cadherin antibody (VE-Cad ab; CAD5, 5 μg ml −1 ) for 6 h. Total cell lysates were analysed by western blotting for phosphorylated and total YAP expression using specific antibodies. The graph represents western blot quantification. ( i ) Immunofluorescence analysis of YAP in VE-Cad antibody-treated HUVECs. ( j ) Intracellular localization of YAP was quantified. Scale bar, 20 μm. Green: YAP, blue: DAPI. ( k ) Densely cultured HUVECs were treated with VE-cadherin antibody (5 μg ml −1 ). Relative level of ANKRD, CTGF and Cyr61 transcript was determined. Data are means±s.d. of triplicates. * P <0.05, ** P <0.01, *** P <0.001 (two-tailed Student’s t -test). Nu, Both, and Cyto indicate the nuclear, both nuclear- and cytoplasmic-, and cytoplasmic-localized YAP, respectively. Full size image VE-cadherin-dependent YAP phosphorylation requires Akt VE-cadherin is known to activate Akt in confluent cells, leading to the phosphorylation and suppression of transcription factors, such as FoxO1, in ECs [8] . Consistent with this result, we found that Akt phosphorylation was reduced by VE-cadherin knockdown or blockade of VE-cadherin clustering ( Fig. 5a,b and Supplementary Fig. 8a,b ). In addition, thrombin reduced Akt phosphorylation ( Fig. 5c,d ). Interestingly, increased Akt phosphorylation was detected in the cytosolic fraction of densely cultured ECs, compared with that in sparse cells ( Supplementary Fig. 8c ), and this correlated with the cytosolic phosphorylation of YAP. Unlike Akt, LATS, an upstream kinase of YAP in the Hippo pathway, did not appear to be activated by VE-cadherin in densely cultured ECs, because the siRNA-mediated depletion of VE-cadherin did not reduce LATS1 phosphorylation ( Supplementary Fig. 9a ). Furthermore, LATS1 phosphorylation was not significantly changed by thrombin in ECs ( Supplementary Fig. 9b ). Although the deficiency or inactivation of LATS1 or LATS2 using siRNAs or the kinase-defective mutant of LATS marginally decreased YAP phosphorylation, it was not enough to induce YAP activation in ECs ( Supplementary Fig. 9c–f ). Because YAP is also a known substrate of Akt [21] , we examined whether blockade of the Akt pathway affects YAP phosphorylation. Both Ly294002, an inhibitor of phosphoinositide 3-kinase (PI3K), and MK-2206, an allosteric inhibitor of Akt, suppressed cell contact-mediated YAP phosphorylation ( Fig. 5e,f and Supplementary Fig. 10 ). In contrast, the Akt inhibitor had no effect on YAP phosphorylation in sparsely cultured cells ( Supplementary Fig. 11a ). In addition, direct suppression of Akt using siRNA or dominant-negative Akt (DN-Akt) inhibited YAP phosphorylation in confluent ECs ( Fig. 5g,h and Supplementary Fig. 11b ). Conversely, overexpression of the constitutively active form of Akt (Myr-HA-Akt) increased YAP phosphorylation in confluent ECs ( Supplementary Fig. 11c ). Interestingly, Myr-HA-Akt expression or serum stimulation in sparse cells did not increase YAP phosphorylation. Instead, YAP phosphorylation was decreased, and its activity was increased ( Supplementary Fig. 12 ), indicating the requirement of cell contact for positive Akt-YAP signalling. The nuclear localization of YAP and the expression of YAP-dependent genes were also increased by Ly294002 in confluent cells, but not in sparse cells ( Fig. 5i,j and Supplementary Fig. 13a,b ). Luciferase assay results also revealed increased transcriptional activity of YAP upon Akt inhibitor treatment or DN-Akt expression ( Fig. 5k and Supplementary Fig. 13c ), indicating the important role of Akt as an upstream kinase of YAP in contacted ECs. Therefore, it is likely that Akt, rather than LATS, is the major kinase in VE-cadherin-induced YAP phosphorylation in ECs. 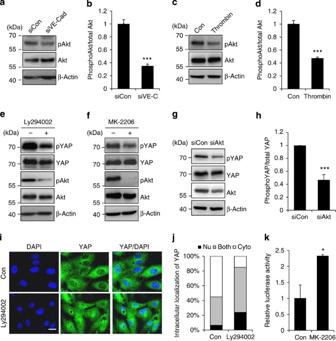Figure 5: VE-cadherin-induced Akt activation mediates YAP phosphorylation and translocation in ECs. (a,b) HUVECs were transfected with control or VE-cadherin siRNA (siVE-Cad) and cultured under dense conditions for 40 h. Cells were starved for 8 h, and phosphorylation of Akt was analysed by western blotting. The graph represents western blot quantification. (c,d) HUVECs were starved for 1 h and treated with thrombin (1 U) for 1 h. Total cell lysates were probed with anti-pAkt, Akt or β-actin antibody. The representative blots of three independent experiments are depicted, and the normalized values for p-Akt are shown. (e) HUVECs were grown to 90% confluence, starved for 24 h and incubated overnight in complete medium with phosphoinositide 3-kinase inhibitor Ly294002 (10 μM). (f) HUVECs were cultured and starved as described as indand incubated for 8 h in complete medium with the Akt inhibitor, MK-2206 (1 μM). pAkt, Akt, pYAP and YAP were detected by western blotting using specific antibodies. (g) HUVECs were transfected with control or Akt siRNA (siAkt) and cultured under confluent conditions for 48 h. Total cell lysates were analysed for YAP phosphorylation by western blotting. (h) Quantification of normalized YAP phosphorylation is shown. (i) Immunofluorescence analysis of YAP in HUVECs treated with Ly294002. (j) Intracellular localization of YAP was quantified. Scale bar, 20 μm. Green: YAP, blue: DAPI. (k) Cells were transfected with p8XGTIIC-luciferase reporter and treated with MK-2206 as described ine. Luciferase activity was measured and normalized to Renilla luciferase activity. Data are means±s.d. of triplicates. ***P<0.0001, *P<0.05 (two-tailed Student’st-test). Figure 5: VE-cadherin-induced Akt activation mediates YAP phosphorylation and translocation in ECs. ( a , b ) HUVECs were transfected with control or VE-cadherin siRNA (siVE-Cad) and cultured under dense conditions for 40 h. Cells were starved for 8 h, and phosphorylation of Akt was analysed by western blotting. The graph represents western blot quantification. ( c , d ) HUVECs were starved for 1 h and treated with thrombin (1 U) for 1 h. Total cell lysates were probed with anti-pAkt, Akt or β-actin antibody. The representative blots of three independent experiments are depicted, and the normalized values for p-Akt are shown. ( e ) HUVECs were grown to 90% confluence, starved for 24 h and incubated overnight in complete medium with phosphoinositide 3-kinase inhibitor Ly294002 (10 μM). ( f ) HUVECs were cultured and starved as described as in d and incubated for 8 h in complete medium with the Akt inhibitor, MK-2206 (1 μM). pAkt, Akt, pYAP and YAP were detected by western blotting using specific antibodies. ( g ) HUVECs were transfected with control or Akt siRNA (siAkt) and cultured under confluent conditions for 48 h. Total cell lysates were analysed for YAP phosphorylation by western blotting. ( h ) Quantification of normalized YAP phosphorylation is shown. ( i ) Immunofluorescence analysis of YAP in HUVECs treated with Ly294002. ( j ) Intracellular localization of YAP was quantified. Scale bar, 20 μm. Green: YAP, blue: DAPI. ( k ) Cells were transfected with p8XGTIIC-luciferase reporter and treated with MK-2206 as described in e . Luciferase activity was measured and normalized to Renilla luciferase activity. Data are means±s.d. of triplicates. *** P <0.0001, * P <0.05 (two-tailed Student’s t -test). Full size image YAP transcriptionally regulates ANG-2 in EC ANG-2, an autocrine factor that is released from active ECs, regulates angiogenesis in a pro- or anti-angiogenic manner, depending on cell context [11] , [13] . Because YAP is localized in the nucleus in loosely contacted ECs, which is a feature of relatively active ECs, we expected that YAP might regulate ANG-2. To test this hypothesis, we reduced or overexpressed YAP in ECs and examined the expression of ANG-2. ANG-2 expression correlated with the expression level of YAP in HUVECs ( Fig. 6a–d and Supplementary Fig. 14a,b ). In agreement with these results, higher ANG-2 expression was detected in sparse cells than in confluent cells ( Supplementary Fig. 14c ). At P8, mouse retinal vessels start invading the deeper vessel layer from the superficial layer. Immunofluorescence staining of mouse retinas (P5 and P8) revealed that ANG-2 protein co-localized with YAP in the front region and invading regions of retinal vessels at P5 and P8, respectively ( Supplementary Fig. 14d and Fig. 6e,f ). ANG-2 is known to be highly expressed in tumour vessels, which are abnormally leaky and tortuous. Yap also co-localized with Ang-2 in tumour vessels ( Supplementary Fig. 14e ), indicating that YAP might be the regulator of ANG-2 in these pathological vessels. To determine how YAP regulates ANG-2, we examined the promoter activity of ANG-2 in ECs. YAP overexpression increased ANG-2 promoter activity ( Fig. 6g ). Chromatin immunoprecipitation analysis of the ANG-2 promoter revealed the binding of YAP to the promoter, thus implying that YAP transcriptionally regulates ANG-2 ( Fig. 6h ). Furthermore, ANG-2 induction by thrombin was suppressed by YAP knockdown ( Fig. 6i ). 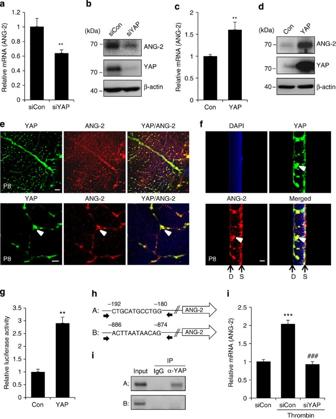Figure 6: YAP regulates ANG-2 expression in ECs. (a,b) HUVECs were transfected with control or YAP siRNA. ANG-2 transcript and protein levels were determined by semi-quantitative reverse transcription–PCR (qRT–PCR) and western blot analysis, respectively. (c,d) Cells were transfected with pCMV2-flag mock or pCMV2-flag-YAP vector (2 μg). ANG-2 mRNA and protein expression were determined by qRT–PCR and western blot analysis, respectively. (e,f) Ang-2 co-localized with Yap protein in mouse retinal vessels. Mouse retinas (P8) were prepared, and immunofluorescence staining was performed using specific antibodies. White arrow heads indicate the co-localization of Yap and Ang-2. Scale bars, 50 μm (upper) and 20 μm (lower). (f) The combined z-stacks are shown vertically. Scale bar, 20 μm. S: superficial layer, D: deeper layer. green: Yap, red: ANG-2, blue: DAPI. (g) HUVECs were transfected with the ANG-2 promoter-Gaussia luciferase reporter vector, along with control or YAP-expressing plasmids. The culture medium was collected 48 h after transfections, and luciferase activity was measured and normalized to secreted alkaline phosphatase activity, which was contained in the reporter vector. Data are means±s.d. of triplicates; **P<0.01 two-tailed Student'st-test. (h) Chromatin immunoprecipitation analysis of the binding of YAP to the ANG-2 promoter was performed. Protein-bound chromatin was prepared from HUVECs and immunoprecipitated with the YAP antibody. Normal IgG was used as a negative control. The immunoprecipitated DNA was analysed by PCR using primers flanking each binding sequence of TEAD (A and B). (i) HUVECs were transfected with control or YAP siRNA and treated with thrombin, as previously described. Total RNA was extracted, and the relative transcript level of ANG-2 was determined by semiquantitative RT–PCR. Data are means±s.d. of triplicates. ***P<0.001 versus control.##P<0.01 versus thrombin treated, control siRNA transfected cells. (two-tailed Student’st-test). These results altogether suggest that YAP is critically involved in the transcriptional regulation of ANG-2 expression in ECs Figure 6: YAP regulates ANG-2 expression in ECs. ( a , b ) HUVECs were transfected with control or YAP siRNA. ANG-2 transcript and protein levels were determined by semi-quantitative reverse transcription–PCR (qRT–PCR) and western blot analysis, respectively. ( c , d ) Cells were transfected with pCMV2-flag mock or pCMV2-flag-YAP vector (2 μg). ANG-2 mRNA and protein expression were determined by qRT–PCR and western blot analysis, respectively. ( e , f ) Ang-2 co-localized with Yap protein in mouse retinal vessels. Mouse retinas (P8) were prepared, and immunofluorescence staining was performed using specific antibodies. White arrow heads indicate the co-localization of Yap and Ang-2. Scale bars, 50 μm (upper) and 20 μm (lower). ( f ) The combined z-stacks are shown vertically. Scale bar, 20 μm. S: superficial layer, D: deeper layer. green: Yap, red: ANG-2, blue: DAPI. ( g ) HUVECs were transfected with the ANG-2 promoter-Gaussia luciferase reporter vector, along with control or YAP-expressing plasmids. The culture medium was collected 48 h after transfections, and luciferase activity was measured and normalized to secreted alkaline phosphatase activity, which was contained in the reporter vector. Data are means±s.d. of triplicates; ** P <0.01 two-tailed Student's t -test. ( h ) Chromatin immunoprecipitation analysis of the binding of YAP to the ANG-2 promoter was performed. Protein-bound chromatin was prepared from HUVECs and immunoprecipitated with the YAP antibody. Normal IgG was used as a negative control. The immunoprecipitated DNA was analysed by PCR using primers flanking each binding sequence of TEAD (A and B). ( i ) HUVECs were transfected with control or YAP siRNA and treated with thrombin, as previously described. Total RNA was extracted, and the relative transcript level of ANG-2 was determined by semiquantitative RT–PCR. Data are means±s.d. of triplicates. *** P <0.001 versus control. ## P <0.01 versus thrombin treated, control siRNA transfected cells. (two-tailed Student’s t -test). Full size image YAP controls vascular remodelling via ANG-2 To investigate the functional relevance of YAP as an ANG-2 regulator in vivo , we injected YAP siRNA into mice at P3 and P4 and analysed retinal vessel development at P5. Injection of siRNA efficiently reduced the expression of YAP mRNA and protein in the mouse retina ( Fig. 7a ). Vascular density and the number of branching points were decreased in Yap siRNA-injected mouse retinas ( Fig. 7b–d ). Similar patterns were also observed in ANG-2-neutralizing antibody-injected mice [22] . Consistently, the mRNA expression of ANG-2 was significantly reduced in Yap siRNA-injected mouse retinas ( Fig. 7e,f ). Furthermore, co-injection with recombinant mouse ANG-2 (rm Ang-2) partially restored Yap siRNA-induced vascular defects ( Fig. 7g,h ), suggesting that YAP plays important roles in postnatal angiogenesis through ANG-2 regulation. 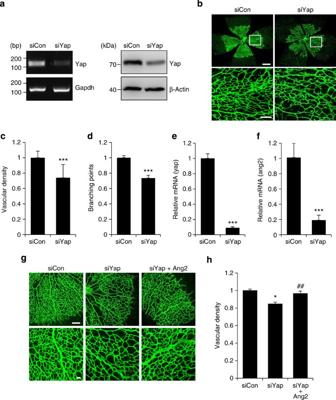Figure 7: YAP regulates angiogenesis via ANG-2in vivo. (a–d) Mice were consecutively injected intraperitoneally with 10 mg kg−1control (siCon) or YAP siRNA (siYap) at P3 and P4. (a) Reverse transcription–PCR (RT–PCR; left) or western blot analysis (right) of Yap expression in retina of mouse injected with siRNA. (b) Mice were killed at P5, and whole-mount retinas were stained with Isolectin-B4. Scale bars, 500 μm (upper) and 50 μm (lower). (c) Quantification of vessel density and (d) branching points are shown. (e,f) Relative mRNA levels of YAP and ANG-2 were measured by real-time RT–PCR. Three mice per group were used. Similar results were obtained from two independent experiments. Data are means±s.e.m.; ***P<0.001 of triplicates (two-tailed Student'st-test). (g,h) Mice were consecutively injected intraperitoneally with 10 mg kg−1control (sicon) or YAP siRNA (siYap) with or without recombinant ang-2 protein (1 mg kg−1) at P3 and P4. Mice were killed at P5, and whole-mount retinas were stained with Isolectin-B4 (g). Scale bars, 200 μm (upper) and 50 μm (lower). (h) Quantification of vessel density. Three mice per group were used. Similar results were obtained from two independent experiments. Data are means±s.e.m.;*P<0.05 versus control cells.##P<0.01 versus untreated siYap transfected cells (two-tailed Student'st-test). GADPH, glyceraldehyde 3-phosphate dehydrogenase. Figure 7: YAP regulates angiogenesis via ANG-2 in vivo . ( a – d ) Mice were consecutively injected intraperitoneally with 10 mg kg −1 control (siCon) or YAP siRNA (siYap) at P3 and P4. ( a ) Reverse transcription–PCR (RT–PCR; left) or western blot analysis (right) of Yap expression in retina of mouse injected with siRNA. ( b ) Mice were killed at P5, and whole-mount retinas were stained with Isolectin-B4. Scale bars, 500 μm (upper) and 50 μm (lower). ( c ) Quantification of vessel density and ( d ) branching points are shown. ( e , f ) Relative mRNA levels of YAP and ANG-2 were measured by real-time RT–PCR. Three mice per group were used. Similar results were obtained from two independent experiments. Data are means±s.e.m. ; *** P <0.001 of triplicates (two-tailed Student's t -test). ( g , h ) Mice were consecutively injected intraperitoneally with 10 mg kg −1 control (sicon) or YAP siRNA (siYap) with or without recombinant ang-2 protein (1 mg kg −1 ) at P3 and P4. Mice were killed at P5, and whole-mount retinas were stained with Isolectin-B4 ( g ). Scale bars, 200 μm (upper) and 50 μm (lower). ( h ) Quantification of vessel density. Three mice per group were used. Similar results were obtained from two independent experiments. Data are means±s.e.m. ; *P <0.05 versus control cells. ## P <0.01 versus untreated siYap transfected cells (two-tailed Student's t -test). GADPH, glyceraldehyde 3-phosphate dehydrogenase. Full size image To further investigate the role of YAP as an ANG-2 regulator in ECs, we examined the effect of YAP on endothelial sprouting using a three-dimensional fibrin gel bead assay. Overexpression of the active form of YAP (YAP S127) in ECs using lentiviruses enhanced ANG-2 expression and increased EC sprouting ( Fig. 8a–d and Supplementary Fig. 15 ). This result is reminiscent to the previous results using ANG-2-overexpressing ECs, which had more sprouting than control cells [23] . Consistently, the supernatant of YAP-overexpressing cells contained increased levels of ANG-2, whereas YAP knockdown reduced ANG-2 in the supernatant ( Supplementary Fig. 15d ). More importantly, the increment of sprouting in active YAP-expressing ECs was blocked by ANG-2 knockdown or soluble Tie-2 treatment ( Fig. 8a–d ). Conversely, the decreased sprouting of YAP-deficient ECs was restored by the addition of recombinant human ANG-2 protein ( Fig. 8e,f ). These data together implicate ANG-2 as an important downstream effector of YAP in regulating angiogenesis. 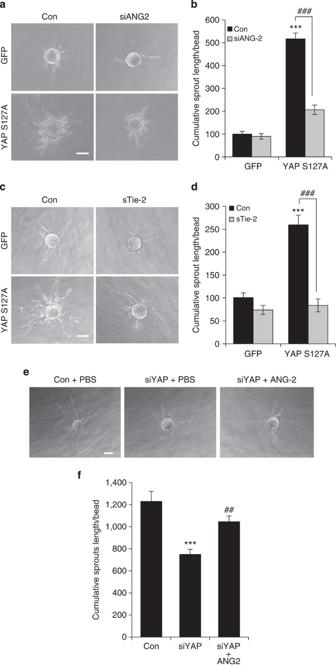Figure 8: YAP controls endothelial sprouting via ANG-2. (a,b) HUVECs were infected with green fluorescent protein (GFP) control (Con) or the YAP S127A-overexpressing lentivirus and subsequently transfected with Con or ANG2 siRNA. The bead-sprouting assay was performed at 16 h after transfection. EGM-2 medium was replaced every other day, and the cumulative sprout length derived per bead was counted after 7 days of incubation. (a) Representative spheroids are shown for each condition. (b) Quantification of cumulative sprout length per bead. (c,d) HUVECs were infected with GFP Con or the YAP S127A-overexpressing lentivirus, and the bead-sprouting assay was performed at 48 h after infection. Con or soluble Tie-2-containing EGM-2 medium (sTie-2, 5 μg ml−1) was replaced every other day, and the cumulative sprout length derived per bead was counted after 7 days of incubation. (c) Representative spheroids are shown for each condition. Scale bar, 100 μm. (d) Quantification of cumulative sprout length per bead. Beads in 25 randomized microscopic fields were counted in each condition. Data represent one experiment. Similar results were obtained from three separate experiments. Data are means±s.e.m. of values from a representative experiment. ***P<0.001 versus GFP-infected Con,###P<0.001 versus untreated YAP S127A-infected cells (two-tailed Student’st-test). (e,f) HUVECs were transfected with Con or YAP siRNA. Fibrin bead sprouting assay was performed in the presence or absence of recombinant human ANG-2 protein (800 ng ml−1) and cumulative sprout length derived from beads was counted after 6 days incubation. (e) Representative spheroids are shown for each condition. Scale bars, 100 μm. (f) Beads in 25 randomized microscopic fields were counted in each condition, and cumulative sprouts length per beads were quantified. Similar results were obtained in three independent experiments. Data were shown as the mean values±s.e.m. of values from a representative experiment.***P<0.0001 versus untreated Con cells.##P<0.01 versus untreated siYAP-transfected cells (two-tailed Student’st-test). Figure 8: YAP controls endothelial sprouting via ANG-2. ( a , b ) HUVECs were infected with green fluorescent protein (GFP) control (Con) or the YAP S127A-overexpressing lentivirus and subsequently transfected with Con or ANG2 siRNA. The bead-sprouting assay was performed at 16 h after transfection. EGM-2 medium was replaced every other day, and the cumulative sprout length derived per bead was counted after 7 days of incubation. ( a ) Representative spheroids are shown for each condition. ( b ) Quantification of cumulative sprout length per bead. ( c , d ) HUVECs were infected with GFP Con or the YAP S127A-overexpressing lentivirus, and the bead-sprouting assay was performed at 48 h after infection. Con or soluble Tie-2-containing EGM-2 medium (sTie-2, 5 μg ml −1 ) was replaced every other day, and the cumulative sprout length derived per bead was counted after 7 days of incubation. ( c ) Representative spheroids are shown for each condition. Scale bar, 100 μm. ( d ) Quantification of cumulative sprout length per bead. Beads in 25 randomized microscopic fields were counted in each condition. Data represent one experiment. Similar results were obtained from three separate experiments. Data are means±s.e.m. of values from a representative experiment. *** P <0.001 versus GFP-infected Con, ### P <0.001 versus untreated YAP S127A-infected cells (two-tailed Student’s t -test). ( e , f ) HUVECs were transfected with Con or YAP siRNA. Fibrin bead sprouting assay was performed in the presence or absence of recombinant human ANG-2 protein (800 ng ml −1 ) and cumulative sprout length derived from beads was counted after 6 days incubation. ( e ) Representative spheroids are shown for each condition. Scale bars, 100 μm. ( f ) Beads in 25 randomized microscopic fields were counted in each condition, and cumulative sprouts length per beads were quantified. Similar results were obtained in three independent experiments. Data were shown as the mean values±s.e.m. of values from a representative experiment. *** P <0.0001 versus untreated Con cells. ## P <0.01 versus untreated siYAP-transfected cells (two-tailed Student’s t -test). Full size image The YAP transcription cofactor is well known to function as an important transcriptional integrator of the Hippo signalling cascade, thereby serving as a transcriptional end point for pathways regulating cell growth, survival and thus organ size [24] . Nuclear localization and activity of YAP, regulated by cellular contact, have been recently reported to control cell proliferation and organ size, and the upstream regulators and downstream targets of YAP are emerging [25] . Considering that junctional stability between ECs is critical in regulating vessel homeostasis and the central importance of ECs in angiogenesis, it is worth investigating the role of YAP in ECs. Furthermore, the physiological relevance of YAP in the vasculature is underscored by a study showing that Yap-deficient mice exhibit defects in yolk sac vasculogenesis [26] . However, its function and significance for the angiogenic activity of ECs has not been demonstrated. We show here for the first time that YAP is highly expressed in ECs and plays a significant role in angiogenesis in vitro and in vivo . We demonstrated that YAP subcellular localization and activity are regulated by VE-cadherin-mediated EC junctions. VE-cadherin-induced YAP phosphorylation is mediated in part by the PI3K-Akt pathway, and YAP subsequently regulates endothelial function through ANG-2. The most well-known function of cell–cell junctions in ECs is to maintain vessel integrity and strictly control the transport of blood proteins and cells between the blood vessels and underlying tissues. However, accumulating evidence suggests that EC junctions play many more roles as signalling structures affecting vascular homeostasis, including contact-induced inhibition of cell growth, apoptosis and new vessel formation. Thus, the modification of endothelial junctional complexes might result in significant changes in vascular permeability, stability and angiogenesis [3] , [4] . The endothelial-specific adhesion protein, VE-cadherin, has emerged as a master regulator of the cell–cell adhesion initiated intracellular signalling pathway. VE-cadherin complexes with p120-catenin and β-catenin at the cell junction to trigger intracellular signalling directly by associating with growth factor receptors or indirectly by regulating gene transcription. Both p120 and β-catenin transcription factors that are released from adhesion complexes by permeability factors such as thrombin are known to translocate to the nucleus and activate target genes [9] . VE-cadherin clustering phosphorylates and suppresses FOXO1 via the PI3K-Akt pathway, leading to the upregulation of claudin-5 expression [8] . Here, we added another transcriptional regulatory mechanism that is triggered by VE-cadherin: VE-cadherin clustering regulates the transcriptional activity of YAP through PI3K-Akt signalling. Several angiogenic factors also activated the PI3K-Akt pathway in ECs, thus raising the issue of signalling specificity. Signalling specificity can be determined by the duration and magnitude of Akt activation. In fact, the possibility of distinct and opposing short-term and long-term consequences of Akt activation in angiogenesis has been raised by several studies [27] , [28] , [29] . Moreover, other signalling molecules, such as ERK, also elicit distinct cellular outcomes depending on the duration and magnitude of their activation [30] . It is conceivable that VE-cadherin clustering can induce relatively low and sustained Akt activation, whereas growth factors can induce robust and transient Akt activation. Thus, differences in the duration and strength of Akt activation may generate variations in signalling output. Low but sustained activation of Akt may play a role by stably phosphorylating YAP to maintain quiescent and stable vessels. Along this line, the role of Akt activation in vessel maturation and stability has been demonstrated in several studies [28] , [31] , [32] . ANG-1, an important cytokine for vessel maturation, activates Akt, leading to the inhibition of vessel destabilization or remodelling genes including ANG-2 (ref. 31 ). Akt1-deficient mice display the impairment of blood vessel maturation and increased vascular permeability [28] . Altogether, our study might be in line with these previous studies, such that Akt activation appears to correlate with vessel stabilization. However, further investigation is needed to determine whether other Akt-activating agents can also phosphorylate YAP through Akt in ECs, and if so, to which extent and for how long. YAP is a downstream transcriptional co-activator of the Hippo pathway that is triggered by cell–cell contact. Despite the significance of cell–cell contact in the regulation of YAP, the upstream cell surface regulators in cell–cell contact-mediated YAP inactivation are still unclear. Alpha-catenin in high-density epithelial cells was found to indirectly bind to YAP via 14-3-3 and thereby inactivate it [19] . The E-cadherin/ β-catenin complex also induces YAP phosphorylation in densely cultured cells and inhibits nuclear accumulation through the Hippo pathway to inhibit cell proliferation [33] . In the present study, knockdown of β-catenin or α-catenin, which is the component of the VE-cadherin junctional complex, reduced YAP phosphorylation in densely cultured ECs ( Supplementary Fig. 7 ). Thus, we added evidence showing that the adherens junction complex is a major upstream regulator of YAP in another cell type, namely ECs. Recently, YAP was demonstrated as an important player in mechanotransduction [16] . Considering the ECs of vessels are exposed to constant haemodynamic flow changes, signal pathways transducing mechanical forces would inevitably exist in ECs. Indeed, adherens junctions composed of VE-cadherin were demonstrated as important mechanical transducers in vascular ECs [34] . Therefore, it would be worthwhile to investigate the functional role of YAP as a mechanosignal transducer in ECs in further studies. Phosphorylation of serine 127 was demonstrated to be important for YAP inactivation and cytoplasmic retention through binding to 14-3-3 (ref. 35 ). LATS is an upstream kinase of YAP in the Hippo kinase cascade pathway [35] . However, we found only marginal changes in YAP phosphorylation following LATS depletion in ECs ( Supplementary Fig. 9 ). Furthermore, VE-cadherin knockdown in ECs did not affect LATS activation ( Supplementary Fig. 9 ), indicating that LATS is unlikely to be the upstream kinase of VE-cadherin-mediated YAP phosphorylation. However, we cannot exclude the possibility that other upstream signalling might induce YAP phosphorylation via LATS in ECs, because LATS knockdown in confluent cells appeared to partially induce translocalization and phosphorylation of YAP in ECs ( Supplementary Fig. 9 ). ANG-2 is known to act as a functional antagonist of ANG-1/Tie-2, and it regulates vascular homeostasis [11] . Although ANG-1 acts constitutively to maintain vessel stability, ANG-2 synthesis and secretion are dynamically regulated. ECs are the primary source of ANG-2 and transcriptionally regulate its production upon activation by cytokines or hypoxia [36] . Furthermore, the secretion of ANG-2 stored in Weibel-Palade bodies of ECs is also tightly regulated [37] . Indeed, thrombin increased both ANG-2 synthesis in ECs and its secretion [38] . However, how ANG-2 is regulated in ECs was not clearly understood, although ANG-2 has been identified as a transcriptional target gene of FOXO1 in ECs [31] , [39] . Interestingly, ANG-2 is also regulated by mechanical shear-stress on ECs. FoxO1 and KLF2 have been shown to play a role in mediating ANG-2 regulation by shear-stress in different ways [40] , [41] . Considering the recent finding that YAP plays a key role in cellular mechanotransduction, it is not surprising that ANG-2 is regulated by YAP in ECs. A recent report showed that ANG-2 transcript levels are inversely correlated with EC density in vitro [22] , thus supporting our hypothesis that ANG-2 may be regulated by cell–cell contact-mediated YAP phosphorylation. Although it is still under investigation how YAP transcriptionally regulates ANG-2, our present study provides new insights into the regulatory mechanism of ANG-2 expression in ECs. In conclusion, we introduced a novel role of YAP as an important angiogenic regulator in ECs. We showed that YAP activity is modulated by the establishment of intercellular junctions mediated by VE-cadherin clustering. Thereby, YAP regulates the endothelial expression of ANG-2, which is important in vascular remodelling and angiogenesis. At the time of angiogenesis, cells emanating from the resting endothelium go through dramatic changes in cell junctions, cytoskeleton and gene expression. However, how and what genes are regulated in those cells has not been clearly defined. The present study suggests that dynamic changes of the subcellular localization of YAP might play a significant role in genetic regulation during endothelial remodelling and sprouting. Furthermore, given that the fine tuning between junctional stability and angiogenic activation of ECs is required for vascular homeostasis, our findings provide important insights into the molecular mechanisms underlying the control of endothelial activation by YAP. Cell culture, antibodies and reagents HUVECs were isolated from human umbilical cord veins by collagenase treatment [42] (Type II, Worthington biochemical Corporation). The vein of cord was washed with warm PBS and filled with pre-warmed collagenase (250 U ml −1 ) and incubated at 37 °C for 10 min. Collagenase solution was collected and centrifuged at 1,000 r.p.m. for 5 min. Pellet was resuspended in 3 ml complete M199 media as described below. HUVECs were grown on plates coated with 2% gelatin in M199 medium (Invitrogen) containing 20% fetal bovine serum (FBS), 100 U ml −1 penicillin, 100 μg ml −1 streptomycin, 3 ng ml −1 basic fibroblast growth factor (R&D Systems) and 5 U ml −1 heparin at 37 °C under a humidified 95%/5% (vol/vol) mixture of air and CO 2 and used at passages 2–7. Transfection of siRNAs and plasmids were performed using Lipofectamine reagent (Invitrogen). Antibodies used in this study were as follows: YAP (Santa Cruz Biotechnology, sc-101199; Cell Signaling, #4912), phospho-YAP (S127, Cell Signaling, #4911), ANG-2 (R&D Systems, MAB0983 or AF623), CDH5 (BD Transduction Laboratories, #610251), Akt (#3787), Phospho-Akt (#9271), LATS1 (#9153), phospho-LATS1 (S909) (#9157; Cell Signaling), LATS2 (Bethyl Laboratories, #A300-479A) and β-actin (Santa Cruz Biotechnology). COMP-ANG-1 was generously provided by Dr Koh [43] . PI3K inhibitor, Ly294002 (L9908), and human thrombin (T7009) were purchased from Sigma. Akt inhibitor, MK-2206, was purchased from Selleckchem (#S1078). Dominant negative Akt (DN Akt) was generously provided by Dr William Sellers (Addgene plasmid #9007) [44] . SiRNA targeting YAP, VE-cadherin, β-catenin or α-catenin was purchased from Dharmacon Inc (On-Target Plus SMARTpool (L-012200-00-0005), (L-003641-00-0005), (L-003482-00-0005) or (L-010505-00-0005)). YAP siRNA was also purchased from Invitrogen (#1062039). For VE-Cadherin, siRNA sequences previously used [45] were also synthesized by Bioneer Inc. (5′-GGAACCAGAUGAACAUUGAUU-3′). Retinal staining Mice were killed by ketamine injection, and eyes were enucleated in PBS. The eyes were fixed in 4% paraformaldehyde (PFA)-PBS (pH 7.4) for 1 h at 4 °C. Retinas were dissected by removing sclera and choroid layer, subsequently the lens, the vitreous humour and hyaloid vessels from the fixed eyes [46] . Retinas were postfixed in 1% PFA-PBS overnight at 4 °C, washed with PBS and permeabilized with PBS containing 1% Triton X-100 for 1 h. Retinas were incubated in blocking solution (Dako) at 4 °C overnight. Retinas were incubated with primary antibodies (YAP, 1:100 and ANG2, 1:100). After washing with PBS, retinas were incubated with Alexa Fluor 488-conjugated goat anti-mouse antibody (1:100) and Alexa Flour 597-conjugated donkey anti-goat antibody (1:100) or Alexa Flour 597-conjugated isolectinGS-IB4 solution (1:100) at 4 °C overnight. Nuclei were stained with 4,6 diamidino-2-phenylindole (DAPI) for 15 min. Flat-mounted retinas were analysed using a confocal fluorescence microscope (LSM 510 META; Carl Zeiss). Fibrin gel bead sprouting assay HUVECs were mixed with dextran-coated Cytodex 3 microcarriers (Amersham Pharmacia Biotech) at a concentration of 400 HUVECs per bead in 1 ml of EGM-2 medium (Clonetics). Beads with cells were shaken gently every 20 min for 4 h at 37 °C and 5% CO 2 . After incubating, beads with cells were transferred to a 25-cm 2 tissue culture flask (BD Biosciences) and left for 12–16 h in 5 ml of EGM-2 at 37 °C and 5% CO 2 . The following day, beads with cells were washed three times with 1 ml EGM-2 and resuspended at a concentration of 250 cell-coated beads per ml in 2 mg ml −1 fibrinogen (Sigma) with 0.15 U ml −1 of aprotinin (Sigma) at a pH of 7.4. Five hundred microlitres of fibrinogen/bead solution was added to 1 unit of thrombin (Sigma) in 1 well of a 24-well tissue culture plate. The fibrinogen/bead solution was allowed to clot for 5 min at room temperature and at 37 °C and 5% CO 2 for 20 min. One millilitre of EGM-2 (which contains 10% FBS) was added to each well and equilibrated with the fibrin clot for 30 min at 37 °C and 5% CO 2 . The medium was removed from the well and replaced with 1 ml fresh medium with or without additional growth factors. Twenty thousand skin fibroblasts were plated on top of the clot, and the medium was changed every other day. Bead assays were monitored for 10 days. Aortic ring assay Aorta was removed from 8-week-old mice and cut into rings ∼ 0.5 mm in width. Five to eight rings were transferred into each well of 24-well plates, incubated in starvation medium for 24 h, and transfected with siRNA using Oligofectamine [46] . Each aortic ring was embedded in fibrin gel in 24-well plates. Embedded rings were fed with Opti-MEM culture medium supplemented with bFGF (basic Fibroblast Growth Factor) to a final concentration of 30 ng ml −1 and 10 μg ml −1 aprotinin. Growth medium was changed first on days 3 or 4 and then changed every other day for a week. Sprouting from aortic rings was quantified at 6–8 days after embedding. Western blot analysis HUVECs were lysed in cell lysis buffer (100 mM Tris-Cl, 5 mM EDTA, 50 mM NaCl, 0.5% NP-40, 1% Triton X-100) containing protease and phosphatase inhibitors. Lysates were centrifuged at 14,000 r.p.m. for 15 min, and the supernatant was collected. Proteins were separated by 8% SDS–polyacrylamide gel electrophoresis and transferred to nitrocellulose membranes. Membranes were incubated with mouse anti-YAP antibody (1;500, Santa Cruz Biotechnology, sc-101199); and goat anti-mouse-HRP (1:5,000, Thermoscientific) was used as the secondary antibody. Detection was performed with ECL Western blotting detection kit (Amersham) according to the manufacturer’s instructions. Images have been cropped for presentation. Full-size images are presented in Supplementary Figs 16–19 . Nuclear and cytoplasmic fraction Cellular fractionation studies were performed on HUVECs cultured in confluent and sparse conditions. After 48 h, cells were washed in cold PBS and lysed with Cyt buffer (10 mM Tris (pH 7.5), 0.05% NP-40, 3 mM MgCl 2 , 100 mM NaCl, 1 mM EGTA, 20 μg ml −1 aprotinin, 1 mM orthovanadate, and 10 μg ml −1 leupeptin). Cells were scrape-loaded into tubes, incubated for 5 min at 4 °C, and spun at 800 g at 4 °C (5 min), and cytosolic supernatants were collected. Cell pellets were further washed with cyto buffer twice to remove residual cytosolic proteins. Purified nuclei were resuspended in SDS-sample buffer as the nuclear fraction. Samples were separated by SDS–polyacrylamide gel electrophoresis and immunoblotted for β-actin and Histone H3 as cytoplasmic and nuclear markers, respectively. Immunofluorescence staining in HUVECs HUVECs cultured on coverslips in a 12-well plate were fixed with 4% PFA-PBS at room temperature for 15 min and permeabilized with 0.1% Triton X-100 in PBS with Tween-20 for 13 min. After blocking with 1% bovine serum albumin in PBS with Tween-20 for 1 h, cells were incubated with anti-YAP antibody (1:100, Santa Cruz Biotechnology, sc-101199) in blocking buffer at 4 °C overnight. After washing with PBS, cells were incubated with Alexa Fluor 488 goat anti-mouse (1:1,000; Molecular Probes) for 1 h at room temperature. Nuclei were stained with DAPI (Molecular Probes). Cells were mounted and images were acquired by a laser scanning confocal microscope (LSM 510 META, Carl Zeiss). More than five microscopic fields were randomly chosen, and cells displaying preferential nuclear YAP localization, even nuclear or cytoplasmic YAP distribution, or cytoplasmic YAP localization were counted. Real-time reverse transcription–PCR (qRT–PCR) For real-time PCR, total RNA (1 μg) isolated from HUVECs using RNeasy (Qiagen) was used for cDNA synthesis by MMLV-RT (Promega Corporation). The abundance of transcripts in the cDNA samples was measured by real-time PCR with specific primers according to the manufacturer’s instructions. The reactions contained Maxima SYBR mix (Thermo Scientific Inc.), 10 pmol of both forward and reverse primers, and cDNA corresponding to 1 μg total RNA. The reactions were subjected to 50 cycles of PCR amplification (95 °C for 10 s, 55 °C for 15 s and 72 °C for 20 s) in a PikoReal 96 (Thermo Scientific Inc.) detection system. All results were normalized to glyceraldehyde 3-phosphate dehydrogenase mRNA. The primers used are described in the Supplementary Table 1 . Luciferase reporter assay HUVECs plated on gelatin-coated dish were transfected with reporter plasmid, p8XGTIIC, a gift of Dr Piccolo (Addgene plasmid #34615) together with internal control vector (pRL-Tk) as described in the figures. Luciferase activity was assayed 24 h after transfection. To examine the effect of thrombin or inhibitors, cells were starved and treated as described in the figure legends. Cells were lysed using a passive lysis buffer (Promega Corporation), and luciferase activity in cell extracts was determined using a dual luciferase assay system following manufacturers’ instructions (Promega Corporation). ANG-2 promoter that was clone-linked to Gaussia luciferase was purchased from GeneCopoeia Inc (Rockville). HUVECs were co-transfected with ANG-2 promoter reporter and YAP and incubated for 48 h. Cell culture medium was collected, and Gaussia luciferase activity was measured following the manufacturer’s protocol (GeneCopoeia Inc.). Lentivirus production Human YAP was cloned into pLenti-C-GFP vector, which was purchased from Origen Technologies. To produce the lentivirus, pLenti-YAP S127A-GFP and 3rd generation packaging DNA were transfected into HEK293t cells. After 48 h, the supernatant was harvested and filtered by a 0.45-μm filter to remove cellular debris. The titration of lentivirus was 10 7 TU per ml. In vivo siRNA injection Mice were injected intraperitoneally with 10 mg kg −1 control or Yap siRNA at P3 and P4 consecutively. Mice were killed at day 5, and the enucleated eyes were processed for retinal whole mount analysis described in Methods (Retinal staining) and stained with Isolectin-B4. Mouse Yap siRNA sequence was selected among four sets of mouse Yap siRNA (Dharmacon On-target plus Smartpool LQ-046247-01-0002) and manufactured as in vivo siSTABLE RNA by Dharmacon Inc. (5′-AAGGAGAGACUGCGGUUGAUU-3′). Statistical analysis Data are presented as mean±standard deviation (s.d.). Statistical comparisons between groups were performed using a two-tailed Student’s t -test. How to cite this article: Choi, H.-J. et al. Yes-associated protein regulates endothelial cell contact-mediated expression of angiopoietin-2. Nat. Commun. 6:6943 doi: 10.1038/ncomms7943 (2015).